Competition for FcRn-mediated transport gives rise to short half-life of human IgG3 and offers therapeutic potential Human IgG3 displays the strongest effector functions of all IgG subclasses but has a short half-life for unresolved reasons. Here we show that IgG3 binds to IgG-salvage receptor (FcRn), but that FcRn-mediated transport and rescue of IgG3 is inhibited in the presence of IgG1 due to intracellular competition between IgG1 and IgG3. We reveal that this occurs because of a single amino acid difference at position 435, where IgG3 has an arginine instead of the histidine found in all other IgG subclasses. While the presence of R435 in IgG increases binding to FcRn at neutral pH, it decreases binding at acidic pH, affecting the rescue efficiency—but only in the presence of H435–IgG. Importantly, we show that in humans the half-life of the H435-containing IgG3 allotype is comparable to IgG1. H435–IgG3 also gave enhanced protection against a pneumococcal challenge in mice, demonstrating H435–IgG3 to be a candidate for monoclonal antibody therapies. Human IgG3 activates complement and FcγR-mediated functions more effectively than any other subclass, followed by IgG1, IgG2 and IgG4, respectively, making it an ideal candidate for immunotherapy [1] , [2] , [3] , [4] . However the short half-life of one week for IgG3, compared with three weeks for the other subclasses, currently makes IgG1 the therapeutic subclass of choice [4] , [5] . The exceptionally long half-life of IgG is mediated by a single receptor, the neonatal Fc receptor for IgG (FcRn) [6] , [7] . FcRn is a heterodimer consisting of a unique MHC class-I like α-chain, associated with β2M. Because its affinity for IgG is negligible at physiological pH ( ∼ 7.4), FcRn binds to IgG only after pinocytosis within early endosomes (pH ≤6.5) [8] , [9] . FcRn–IgG complexes are then routed away from the lysosomal pathway [10] , [11] , [12] , [13] , and either cycled back to the cell surface or transported to the opposite side of the cell. The vesicles fuse with the plasma membrane, returning the pH to ∼ 7.4, and releasing IgG [14] , [15] , [16] . Besides IgG transport, FcRn enhances IgG-mediated phagocytosis as well as antigen presentation by both MHC class I and II [16] , [17] , [18] , [19] , and has a key role in rescuing albumin from lysosomal degradation [20] . Two theoretical explanations for the reduced half-life of IgG3 have been suggested. First, the long hinge region of IgG3 might make it more prone to proteolytic degradation [4] . Second, the recycling of IgG3 by FcRn may be less efficient because of an amino acid difference at position 435—a key contact residue with FcRn and, in IgG1, IgG2 and IgG4, important for the pH-dependent formation of IgG–FcRn complexes through histidine protonation around pH ≤6.5 (refs 8 , 9 , 21 , 22 ). IgG3 contains an arginine in this position (R435), and although both residues classify as positively charged, arginines, unlike histidines, do not deprotonate at neutral pH, theoretically resulting in IgG3 binding to FcRn being less pH-dependent, leading to shortened half-life as described for various mutated IgG variants with increased affinity to FcRn at neutral pH (refs 8 , 23 ). Previous experimental work indeed pointed to the involvement of R435, as human IgG1–Fc and scFv–IgG1–Fc fragments bearing R435 showed reduced half-life in wild-type mice [24] , [25] . Human H435R–IgG4 variant was also reported to display an altered binding to rat FcRn [8] . However, species-incompatible FcRn were used in these studies; the exceptional long hinge of IgG3 was not present; and the underlying mechanisms were not explored [4] , [8] , [24] , [25] , [26] , [27] . Here we investigate the difference in FcRn-mediated transport and rescue of IgG1 and IgG3. Using human in vitro and in vivo models, we observed—unexpectedly—that both IgG1 and IgG3 show pH-dependent binding to FcRn, and that FcRn can transport IgG3 as efficiently as IgG1. However, when both IgG1 and IgG3 are present, IgG1 inhibits FcRn-mediated IgG3 transport, leading to degradation of IgG3. Our data provide strong evidence that the presence of an arginine at position 435 in IgG3 is sufficient to explain its high rate of catabolism observed in vivo . Importantly, we show that the half-life of the H435-containing IgG3 allotype is comparable to IgG1 in humans. Using a mouse model for pneumococcal pneumonia, we provide a proof of concept that IgG3–R435H can be utilized for IgG-based immunotherapies aiming at maximizing effector functions. IgG1 interferes with IgG3 transport To study FcRn-mediated functions, we developed an in vitro transport model by transducing the FcRn-negative human cell line A375 with the human FcRn α-chain (A375–FcRn). The wild-type A375 did not transport IgG using intravenous immunoglobulin (IVIg), a polyclonal mixture of all human IgG subclasses ( Fig. 1a ). However, active transport was observed in A375–FcRn cells in medium buffered at pH 7.4. We found IgG transport in A375–FcRn to be similar to that observed across placental syncytiotrophoblast derived JAR cells expressing endogenous FcRn ( Fig. 1b ). From IVIg, A375–FcRn cells transported IgG3 less effectively than IgG1, but JAR transported relatively equal amounts of both IgG1 and IgG3 ( Fig. 1a,b ). 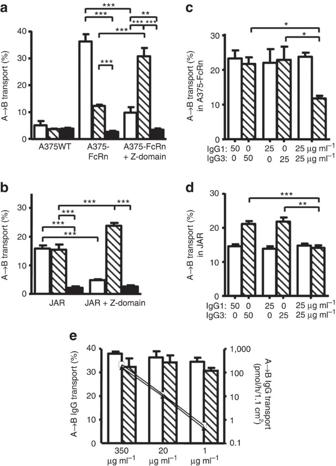Figure 1: IgG3 transport is inhibited by IgG1 at non-saturating conditions. All experiments were performed at pH 7.4. (a) FcRn-negative human A375-WT cells did not transcytose IgG1 (white) and IgG3 (hatched) from IVIg as transport was comparable to passive leakage (HRP, black). After transfection with the FcRn α-chain, A375–FcRn efficiently transported IgG from the apical to the basolateral compartment. When IVIg was mixed with Z-domain before transport at a 2:1 molar ratio (Z-domain:IgG) the IgG1 transport by A375–FcRn cells was significantly reduced, while IgG3 transport was enhanced. (b) JAR cells naturally expressing FcRn transported IgG1 and IgG3 from IVIg equally well. Incubation of IVIg with the Z-domain at a 2:1 molar ratio before transport inhibited transport of IgG1 but increased transport of IgG3. (c) Purified IgG3 and IgG1 were transcytosed equally well in A375–FcRn cells when transported separately, and neither inhibited its own transport when the input was doubled. Yet in 1:1 mixtures, IgG3 transport was reduced in the presence of IgG1. (d) In JAR cells, IgG3 was efficiently transported when offered alone. The amount of either IgG1 or IgG3 transported was also unaffected by doubling the apical concentration, but IgG3 transport was inhibited by the presence of equal amounts of IgG1. (e) When only one subclass was present, A375–FcRn transported a fixed percentage of IgG (left axis), while the absolute amount transported was diminished (IgG1 open squares, IgG3 triangles, right axis). Throughout, IgG1 is represented by open bars, IgG3 by hatched bars. 100 μg ml−1IVIg was used in both (a,b). Apical to basolateral transport of myeloma IgG1 and IMIg-derived IgG3 in the concentration indicated in (c–e). TheY-axis represents the percentage of IgG transported from the apical compartment to the basolateral compartment. The data represent mean and standard deviation from three independent experiments. Statistical comparison was performed by one-way ANOVA followed by Tukey's multiple comparison test in (a,b), and transport of IgG3, in the presence of IgG1, was compared with transport of IgG3 alone by two-tailedt-test in (c,d). *P≤0.05; **P≤0.01; ***P≤0.001. Figure 1: IgG3 transport is inhibited by IgG1 at non-saturating conditions. All experiments were performed at pH 7.4. ( a ) FcRn-negative human A375-WT cells did not transcytose IgG1 (white) and IgG3 (hatched) from IVIg as transport was comparable to passive leakage (HRP, black). After transfection with the FcRn α-chain, A375–FcRn efficiently transported IgG from the apical to the basolateral compartment. When IVIg was mixed with Z-domain before transport at a 2:1 molar ratio (Z-domain:IgG) the IgG1 transport by A375–FcRn cells was significantly reduced, while IgG3 transport was enhanced. ( b ) JAR cells naturally expressing FcRn transported IgG1 and IgG3 from IVIg equally well. Incubation of IVIg with the Z-domain at a 2:1 molar ratio before transport inhibited transport of IgG1 but increased transport of IgG3. ( c ) Purified IgG3 and IgG1 were transcytosed equally well in A375–FcRn cells when transported separately, and neither inhibited its own transport when the input was doubled. Yet in 1:1 mixtures, IgG3 transport was reduced in the presence of IgG1. ( d ) In JAR cells, IgG3 was efficiently transported when offered alone. The amount of either IgG1 or IgG3 transported was also unaffected by doubling the apical concentration, but IgG3 transport was inhibited by the presence of equal amounts of IgG1. ( e ) When only one subclass was present, A375–FcRn transported a fixed percentage of IgG (left axis), while the absolute amount transported was diminished (IgG1 open squares, IgG3 triangles, right axis). Throughout, IgG1 is represented by open bars, IgG3 by hatched bars. 100 μg ml −1 IVIg was used in both ( a , b ). Apical to basolateral transport of myeloma IgG1 and IMIg-derived IgG3 in the concentration indicated in ( c – e ). The Y -axis represents the percentage of IgG transported from the apical compartment to the basolateral compartment. The data represent mean and standard deviation from three independent experiments. Statistical comparison was performed by one-way ANOVA followed by Tukey's multiple comparison test in ( a , b ), and transport of IgG3, in the presence of IgG1, was compared with transport of IgG3 alone by two-tailed t -test in ( c , d ). * P ≤0.05; ** P ≤0.01; *** P ≤0.001. Full size image When IVIg was pre-incubated with Z-domains of protein A, a selective competitive inhibitor of FcRn binding to IgG1, IgG2 and IgG4 (refs 28 , 29 ), transport of IgG1 by JAR and A375–FcRn cells was reduced to levels approaching those found in parental A375-WT and for non-specific horseradish peroxidase (HRP) transport and ( Fig. 1 ), indicating IgG1 transport to be FcRn-dependent in both cell types. Remarkably, IgG3 transport was significantly increased in both JAR and A375–FcRn cells by the addition of Z-domains ( Fig. 1a,b ), suggesting that active transport of the other IgG subclasses interfered with IgG3 transport. We therefore studied the effect of IgG1 on the FcRn-mediated transport of IgG3 using purified antibodies. Indeed, IgG3 alone was transported equally well as IgG1, and the transport of IgG3 was inhibited by adding IgG1 to A375–FcRn ( Fig. 1c ) or JAR cells ( Fig. 1d ). As the percentage of IgG1 or IgG3 transport was unaffected by the initial IgG concentration (measured over a range from 1 to 350 μg ml −1 ; Fig. 1e ) the observed inhibition of IgG3 transport by IgG1 (at concentrations of 50–100 μg ml −1 ) cannot be owing to FcRn saturation. The pH in the extracelluar medium was set at pH 7.4, suggesting the inhibition to takes place in intracellular compartments. IgG1 and IgG3 compete for binding to FcRn and transport Ober et al . demonstrated that, during sorting, the unbound FcRn molecules are routed away from the sorting endosomes [15] . This might explain the observed competition between IgG1 and IgG3 for FcRn binding and transport, because the number of FcRn molecules in intracellular compartments can also become limited under non-saturating conditions. Indeed, we show that when the IgG3 concentration was kept constant at 10 μg ml −1 , IgG1 concentrations as low as 1 ng ml −1 significantly reduced IgG3 transport ( Fig. 2a ). When IgG1 and IgG3 were mixed in equal amounts, the relative IgG3 transport was significantly reduced, compared with transport of IgG3 alone at high concentrations, but was unaffected at IgG concentrations of 10 ng ml −1 /subclass, when ∼ 4% of 1.25 μm sorting endosomes [15] would be expected to contain IgG ( Fig. 2b ). Remarkably, this concentration of IgG1 (10 ng ml −1 ) significantly inhibited a 1,000-fold excess of IgG3 (10 μg ml −1 , Fig. 2a ). Similarly, soluble IgG1 was more efficient than IgG3 in inhibiting binding of soluble human FcRn (shFcRn) to IgG3-immobilized biosensor chips ( Fig. 2c,d ). 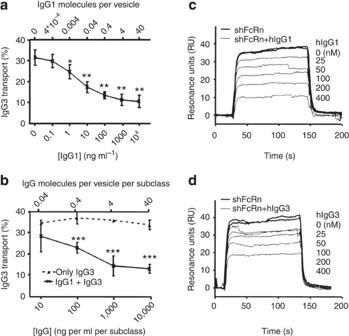Figure 2: Concentration-dependent inhibition of IgG3 transport by IgG1 owing to competitive binding to FcRn. Apical to basolateral transport of V-gene matched recombinant IgG3 and IgG1. (a) IgG3 concentration was kept constant (10 μg ml−1) in the absence or presence of increasing amounts of IgG1. IgG3 transport was inhibited up to a plateau when more than 1 ng ml−1IgG1 was present. All data points were compared with the samples without IgG1 by one-way ANOVA and Dunnett's multiple comparison test. (b) Recombinant IgG3 alone (dotted line) or mixed with IgG1 (solid line) at a 1:1 ratio in increasing concentrations were added to the apical compartment and IgG3 was measured in the basolateral compartment. At concentrations lower than 1 μg ml−1, transport of IgG3 increased up to levels similar to those observed when IgG3 is transported alone. All data points from mixed IgG1 and IgG3 transport in (b) were compared byt-test to the corresponding IgG3 transport without IgG1 present. The theoretical number of IgG molecules present in 1.25-μm-wide sorting endosomes described in ref.15, assuming an equal concentration within these vesicles as present in the medium, is indicated on the secondary upperx-axis in (a,b). This arbitrary value is given as an indication only as these calculated values cannot take miscellaneously elongated or tubule-tethered vesicles into account13,15(c,d). Surface plasma resonance analysis showing binding of 100-nM recombinant shFcRn to IgG3-immobilized CM5 biosensor chips (1,300 RU) at pH 6.0 in the presence of increasing concentrations of 25, 50, 100, 200 or 400-nM recombinant soluble IgG1 (c) or IgG3 (d). The data in (a,b) represent the mean and standard deviation. All experiments were repeated at least three times with similar results. *P≤0.05; **P≤0.01; ***P≤0.001. Figure 2: Concentration-dependent inhibition of IgG3 transport by IgG1 owing to competitive binding to FcRn. Apical to basolateral transport of V-gene matched recombinant IgG3 and IgG1. ( a ) IgG3 concentration was kept constant (10 μg ml −1 ) in the absence or presence of increasing amounts of IgG1. IgG3 transport was inhibited up to a plateau when more than 1 ng ml −1 IgG1 was present. All data points were compared with the samples without IgG1 by one-way ANOVA and Dunnett's multiple comparison test. ( b ) Recombinant IgG3 alone (dotted line) or mixed with IgG1 (solid line) at a 1:1 ratio in increasing concentrations were added to the apical compartment and IgG3 was measured in the basolateral compartment. At concentrations lower than 1 μg ml −1 , transport of IgG3 increased up to levels similar to those observed when IgG3 is transported alone. All data points from mixed IgG1 and IgG3 transport in ( b ) were compared by t -test to the corresponding IgG3 transport without IgG1 present. The theoretical number of IgG molecules present in 1.25-μm-wide sorting endosomes described in ref. 15 , assuming an equal concentration within these vesicles as present in the medium, is indicated on the secondary upper x -axis in ( a , b ). This arbitrary value is given as an indication only as these calculated values cannot take miscellaneously elongated or tubule-tethered vesicles into account [13] , [15] ( c , d ). Surface plasma resonance analysis showing binding of 100-nM recombinant shFcRn to IgG3-immobilized CM5 biosensor chips (1,300 RU) at pH 6.0 in the presence of increasing concentrations of 25, 50, 100, 200 or 400-nM recombinant soluble IgG1 ( c ) or IgG3 ( d ). The data in ( a , b ) represent the mean and standard deviation. All experiments were repeated at least three times with similar results. * P ≤0.05; ** P ≤0.01; *** P ≤0.001. Full size image R435 in IgG interferes with binding to FcRn When the differences in position 435 between IgG1 (Histidine) and IgG3 (Arginine) were modelled into the existing crystal structure [21] , it was clear that the longer side chain of arginine may potentially disrupt the tight fit of IgG in the FcRn-binding pocket ( Fig. 3a,b ). However, theoretically it may also convey a more favourable charge at pH 7.4, at which the net charge of histidine is neutral but arginine is positive [22] . IgG3 did indeed bind to shFcRn significantly better at pH 7.4, but IgG1 bound better at pH 6.0 as measured by ELISA ( Supplementary Fig. S1 ) and by surface plasmon resonance (SPR) ( Fig. 3c,d ). We subsequently mutated IgG1 to include the IgG3-derived arginine residue and vice versa (IgG1–H435R and IgG3–R435H, respectively). These mutations resulted in the loss (IgG1–H435R) or gain (IgG3–R435H) of protein A binding ( Supplementary Fig. S1 ). 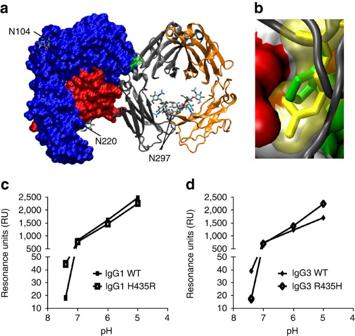Figure 3: The influence of the Histidine versus Arginine at position 435 on FcRn binding at different pH. (a) The crystal structure of FcRn with IgG–Fc part, showing the orientation of the amino acid 435 of IgG in yellow.N-linked glycans are labelled according to their occurrence in FcRn and Fc. (b) A close-up showing the side chain of amino acid 435 of IgG (histidine, in green) in the binding pocket of FcRn. When arginine (present at this position in IgG3) was modelled into this position (yellow), it protrudes into the FcRn surface area (non-polar residues in white, positively charged amino acids in blue, negatively charged residues in red and polar residues in green), suggesting steric hindrance. Histidine at this position alters its charge at pH 6.5 and lower (positive charge, resulting in FcRn binding) versus neutral pH (no charge, resulting in release of IgG from FcRn)22. Arginine in this position, however, is positively charged at both low and neutral pH, possibly resulting in better binding of IgG3 at neutral pH. The crystallographic coordinates51(accession 1I1A) were modelled using DeepView 4.03 (ref.52) and VMD 1.9 (ref.53). (c,d) The importance of this amino acid difference between IgG1 and IgG3 was tested biochemically by injecting 500 nM recombinant IgG over shFcRn-coupled CM5 sensor chips at different pH. IgG3 (d) bound FcRn better than IgG1 (c) at neutral pH, but the situation was reversed at acidic pH. IgG1–H435R mutant gained IgG3-like characteristics, binding better at neutral pH, but worse at low pH (c). Likewise, IgG3 behaved like IgG1 after replacing the R435 with H435, binding relatively worse at neutral pH, but better at low pH (d), confirming that two opposing factors (steric hindrance versus charge) may contribute to the observed inhibition by IgG1 on FcRn-mediated IgG3 transport. The data in (c,d) are presented as individual data points connecting the means from two independent injections with a line. Figure 3: The influence of the Histidine versus Arginine at position 435 on FcRn binding at different pH. ( a ) The crystal structure of FcRn with IgG–Fc part, showing the orientation of the amino acid 435 of IgG in yellow. N -linked glycans are labelled according to their occurrence in FcRn and Fc. ( b ) A close-up showing the side chain of amino acid 435 of IgG (histidine, in green) in the binding pocket of FcRn. When arginine (present at this position in IgG3) was modelled into this position (yellow), it protrudes into the FcRn surface area (non-polar residues in white, positively charged amino acids in blue, negatively charged residues in red and polar residues in green), suggesting steric hindrance. Histidine at this position alters its charge at pH 6.5 and lower (positive charge, resulting in FcRn binding) versus neutral pH (no charge, resulting in release of IgG from FcRn) [22] . Arginine in this position, however, is positively charged at both low and neutral pH, possibly resulting in better binding of IgG3 at neutral pH. The crystallographic coordinates [51] (accession 1I1A) were modelled using DeepView 4.03 (ref. 52 ) and VMD 1.9 (ref. 53 ). ( c , d ) The importance of this amino acid difference between IgG1 and IgG3 was tested biochemically by injecting 500 nM recombinant IgG over shFcRn-coupled CM5 sensor chips at different pH. IgG3 ( d ) bound FcRn better than IgG1 ( c ) at neutral pH, but the situation was reversed at acidic pH. IgG1–H435R mutant gained IgG3-like characteristics, binding better at neutral pH, but worse at low pH ( c ). Likewise, IgG3 behaved like IgG1 after replacing the R435 with H435, binding relatively worse at neutral pH, but better at low pH ( d ), confirming that two opposing factors (steric hindrance versus charge) may contribute to the observed inhibition by IgG1 on FcRn-mediated IgG3 transport. The data in ( c , d ) are presented as individual data points connecting the means from two independent injections with a line. Full size image Using shFcRn-coupled biosensor chips in SPR experiments, we noted that IgG1–H435R showed improved binding to FcRn at pH 7.4 compared with WT IgG1, but reduced binding affinity at acidic pH. Likewise, binding of IgG3–R435H was reduced at pH 7.4, but improved at acidic pH compared with WT IgG3 ( Fig. 3c,d ). The relative binding of both IgG subclasses and variants was however very weak at pH 7.4, but increased steadily as the pH decreased, showing that shFcRn binding remained pH-dependent for all variants. The H435-containing IgG variants bound shFcRn with similar calculated affinities at pH 6.0 according to the bivalent ligand-binding model. However, IgG3 and IgG1–H435R had calculated kinetic dissociation constant (K D s) that were, respectively, two times and ∼ 50% higher than WT IgG1 ( Supplementary Fig. S2 ; Supplementary Table S1 ). Similar results were found using the heterogeneous ligand-binding model and by repeating the experiments with a reversed set-up, using IgG-coupled biosensor chips and the steady-state affinity model [30] : shFcRn bound the strongest to IgG1-coupled chips at pH 6.0 whereas IgG1–H435R showed reduced binding. The affinity of shFcRn was improved for IgG3–R435H compared with IgG3 that showed the weakest affinity of all variants ( Fig. 4 ). 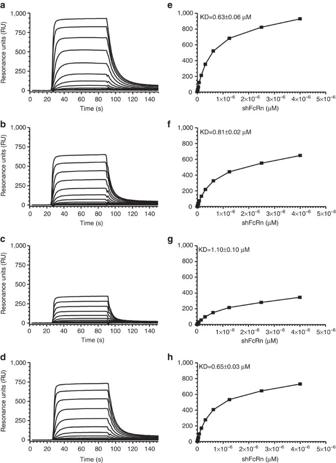Figure 4: Binding of the IgG at pH 6. 0 is influenced by the amino acid at position 435. The different IgG variants (IgG1, IgG1–H435R, IgG3, or IgG3–R435H) were immobilized to CM5 sensor chips and shFcRn injected at different concentrations (7–4,000 nM represented by different lines) at pH 6.0. The sensorgrams are shown in the left panels (a–d), and the corresponding equilibrium-binding responses versus shFcRn concentrations in the right panels (e–h), for IgG1 (a,e), IgG1–H435R (b,f), IgG3 (c,g), or IgG3–R435H (d,h). The calculated affinity constants are superimposed in the right panels as derived from steady-state binding model using the BIAevaluation software. FcRn shows a reduced affinity to IgG1 at pH 6.0 after mutating the H at position 435 to R, and enhanced affinity to IgG3 after mutating the R at position 435 to H. The data are representative from two independent injections. Figure 4: Binding of the IgG at pH 6. 0 is influenced by the amino acid at position 435. The different IgG variants (IgG1, IgG1–H435R, IgG3, or IgG3–R435H) were immobilized to CM5 sensor chips and shFcRn injected at different concentrations (7–4,000 nM represented by different lines) at pH 6.0. The sensorgrams are shown in the left panels ( a – d ), and the corresponding equilibrium-binding responses versus shFcRn concentrations in the right panels ( e – h ), for IgG1 ( a , e ), IgG1–H435R ( b , f ), IgG3 ( c , g ), or IgG3–R435H ( d , h ). The calculated affinity constants are superimposed in the right panels as derived from steady-state binding model using the BIAevaluation software. FcRn shows a reduced affinity to IgG1 at pH 6.0 after mutating the H at position 435 to R, and enhanced affinity to IgG3 after mutating the R at position 435 to H. The data are representative from two independent injections. Full size image The inhibition of IgG3 transport by IgG1 is due to R435 In agreement with the retained pH-dependent FcRn-binding, the presence of histidine or arginine at position 435 did not influence the transport efficiency of either subclass when transported individually in A375–FcRn cells ( Fig. 5a ). When the amino acid at position 435 was mutated to an alanine, binding to protein A and shFcRn ( Supplementary Fig. S1 ) as well as FcRn-dependent transport ( Fig. 5a ), was almost entirely abrogated both for IgG1 and IgG3. When mixed, IgG1–H435A did not inhibit transport of IgG3 ( Fig. 5b ), indicating that binding of IgG1 to FcRn was required for the observed inhibition of IgG3 transport. Importantly, IgG1–H435R ( Fig. 5a ) was also unable to inhibit IgG3 transport ( Fig. 5b ), indicating the arginine/histidine difference between IgG3 and IgG1 to be important for IgG1-mediated inhibition of IgG3 transport. In line with this, transport of IgG3–R435H was unaffected by the presence of any IgG1 variant ( Fig. 5c ). Remarkably, IgG3–R435H inhibited transport of IgG1–H435R ( Fig. 5c ) to a similar extent as IgG1-WT inhibited transport of IgG3-WT ( Fig. 5b ). These results demonstrate that IgG–R435 can be transported by FcRn through cells, but that binding to, and transport by, FcRn is inhibited in the presence of H435-containing IgG. 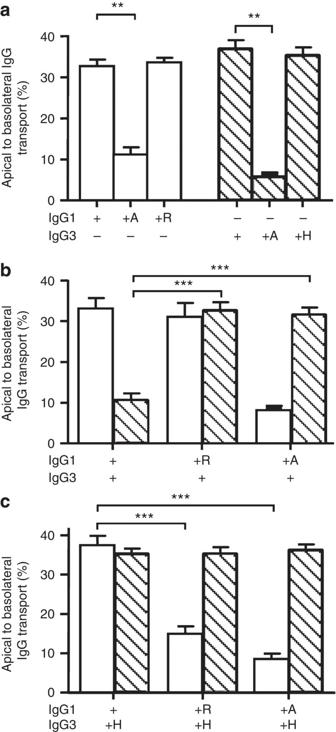Figure 5: Inhibition of IgG3 transport by IgG1 is due to R435 in IgG3. (a) Mutating the amino acid at position 435 in IgG1 (H435) and in IgG3 (R435) to an alanine reduces transport, while exchanging the histidine native to IgG1 and the arginine native to IgG3 on each others backbone had no effect on their transport rate when offered separately to FcRn-transfected A375 cells. (b) Whereas transport of IgG3-WT was inhibited in the presence of IgG1-WT, IgG1 bearing an alanine or an arginine at position 435 had no effect on IgG3 transport. (c) Transport of IgG3 with a histidine at position 435 was not inhibited by WT IgG1. When the amino acids found at position 435 in IgG1 and IgG3 were swapped, IgG1–H435R transport was inhibited by IgG3–R435H. (a–c) ± indicate the presence or absence of IgG (10 μg ml−1per subclass), IgG1 is represented by open bars, IgG3 by hatched bars. The presence of mutated variants (435H, 435A and 435R) is indicated by the corresponding letter. The data represent mean and standard deviation from three independent experiments. Transport of WT IgG was compared with transport of mutant IgG by one-way ANOVA with Dunnett's multiple comparison test and significance. **P≤0.01; ***P≤0.001. Figure 5: Inhibition of IgG3 transport by IgG1 is due to R435 in IgG3. ( a ) Mutating the amino acid at position 435 in IgG1 (H435) and in IgG3 (R435) to an alanine reduces transport, while exchanging the histidine native to IgG1 and the arginine native to IgG3 on each others backbone had no effect on their transport rate when offered separately to FcRn-transfected A375 cells. ( b ) Whereas transport of IgG3-WT was inhibited in the presence of IgG1-WT, IgG1 bearing an alanine or an arginine at position 435 had no effect on IgG3 transport. ( c ) Transport of IgG3 with a histidine at position 435 was not inhibited by WT IgG1. When the amino acids found at position 435 in IgG1 and IgG3 were swapped, IgG1–H435R transport was inhibited by IgG3–R435H. ( a – c ) ± indicate the presence or absence of IgG (10 μg ml −1 per subclass), IgG1 is represented by open bars, IgG3 by hatched bars. The presence of mutated variants (435H, 435A and 435R) is indicated by the corresponding letter. The data represent mean and standard deviation from three independent experiments. Transport of WT IgG was compared with transport of mutant IgG by one-way ANOVA with Dunnett's multiple comparison test and significance. ** P ≤0.01; *** P ≤0.001. Full size image Competition for FcRn leads to degradation of IgG3 in vitro We next tested whether the reduced IgG3 transport in the presence of IgG1 was reflected in enhanced degradation during apical to basolateral transport. We therefore measured the recovery of different IgG variants from the apical and basolateral compartments ( Fig. 6a ). Up to 95% of IgG1 or IgG3 could be accounted for when transported alone. When mixed with IgG3, IgG1 recovery was unaffected, but only 60% of the initial amount of IgG3 was detected. However, when WT IgG1 and IgG3–R435H were mixed, recovery of both was ∼ 95% ( Fig. 6a ), indicating that the decreased transport and enhanced loss of IgG3 in the presence of IgG1 was solely due to the arginine at position 435. 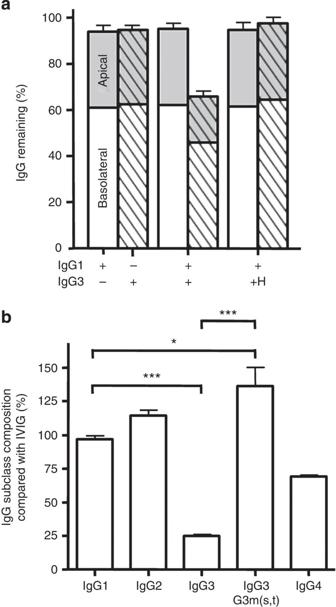Figure 6: H435-containing IgG3 has extended half-life in humans. (a) Approximately 95% of the total IgG added to apical compartments of confluent A375–FcRn monolayers was recovered after 24 h from both the apical (grey) and the basolateral (white) compartments when the IgG1 (open bars) or IgG3 (hatched) were added individually (10 μg ml−1per subclass). However, when the IgG1 and IgG3 were mixed in equal amounts,∼65% of the initial IgG3 could be detected, suggesting IgG3 was degraded in the presence of IgG1. IgG1 recovery was similar to that found when no IgG3 was present. IgG3–R435H was not degraded in the presence of IgG1 as about 95% could be detected after 24 h, similarly to IgG3 alone. The data represent mean and standard deviation from three independent experiments. (b) The relative concentration of IgG subclasses and the histidine-435 containing IgG3 allotype G3m(s,t) in sera from agammaglobulinemic patients four weeks after their last treatment with IVIg compared with IgG subclass and G3m(s,t) levels found in the corresponding IVIg preparation. Data represent the average plus standard deviation calculated from at least three independent IgG subclass and allotype measurements performed on serum from three patients in (b). Statistical comparison was performed by one-way ANOVA followed by Tukey's multiple comparison test in (b). *P≤0.05; ***P≤0.001. For simplicity, significant differences are only displayed for IgG1 compared with all subclasses, and between IgG3 total and G3m(s,t) levels in (b). Figure 6: H435-containing IgG3 has extended half-life in humans. ( a ) Approximately 95% of the total IgG added to apical compartments of confluent A375–FcRn monolayers was recovered after 24 h from both the apical (grey) and the basolateral (white) compartments when the IgG1 (open bars) or IgG3 (hatched) were added individually (10 μg ml −1 per subclass). However, when the IgG1 and IgG3 were mixed in equal amounts, ∼ 65% of the initial IgG3 could be detected, suggesting IgG3 was degraded in the presence of IgG1. IgG1 recovery was similar to that found when no IgG3 was present. IgG3–R435H was not degraded in the presence of IgG1 as about 95% could be detected after 24 h, similarly to IgG3 alone. The data represent mean and standard deviation from three independent experiments. ( b ) The relative concentration of IgG subclasses and the histidine-435 containing IgG3 allotype G3m( s , t ) in sera from agammaglobulinemic patients four weeks after their last treatment with IVIg compared with IgG subclass and G3m( s , t ) levels found in the corresponding IVIg preparation. Data represent the average plus standard deviation calculated from at least three independent IgG subclass and allotype measurements performed on serum from three patients in ( b ). Statistical comparison was performed by one-way ANOVA followed by Tukey's multiple comparison test in ( b ). * P ≤0.05; *** P ≤0.001. For simplicity, significant differences are only displayed for IgG1 compared with all subclasses, and between IgG3 total and G3m( s , t ) levels in ( b ). Full size image IgG3 with H435 has an enhanced half-life in humans The IgG3 G3m( s , t ) allotype ( Supplementary Fig. S3 ) contains a histidine at position 435, and can therefore be used to investigate the in vivo effect of the mutation. Although not commonly found in native Europeans, we found detectable levels in IVIg ( Supplementary Fig. S4 ). [31] , [32] , [33] , [34] We therefore investigated whether R435 can also cause the fast clearance of IgG3 in vivo , by analysing the serum persistence of this IgG3 allotype in sera of IVIg-treated X-linked agammaglobulinemic patients. Compared with the amounts found in the IVIg preparation itself, the amount of IgG1 and IgG2 relative to total IgG was unchanged in these patients four weeks after the last infusion of IVIg ( Fig. 6b ). As expected, the total serum IgG3 level, consisting mostly of R435 containing G3m(b) and G3m(g) allotypes in Europe [31] , [32] ( Supplementary Fig. S3 ), was significantly lowered, but significantly increased for the H435-containing IgG3 allotype G3m( s , t ) ( Fig. 6b ). Thus, also in natural variants of IgG3, the presence of a histidine or an arginine at position 435 determines the catabolic rate in vivo . Enhanced effector functions of H435 containing IgG3 in vivo IgG3 binds C1q and activates FcγR more potently than any of the other IgG subclasses, but its therapeutic application has not yet been considered a viable option because of its short half-life [4] , [35] , [36] . We therefore compared the potential of the recombinant V-gene-matched IgG1, IgG3, IgG1–H435R and IgG3–R435H (directed against Streptococcus pneumoniae serotype 6) [17] , [37] to stimulate FcγR-mediated phagocytosis and mediate protection against pneumococcal pneumonia and bacteremia. IgG3 mediated more phagocytosis than IgG1, and neither isoallotypic alteration (IgG1 H435R/IgG3 R435H) significantly changed the capacity of the antibodies to mediate phagocytosis of pneumococci ( Supplementary Fig. S5 ). We then passively immunized outbred NMRI mice 48 h before measuring the level of the human antibodies and intranasal challenge with virulent pneumococci. The serum persistence of all four IgG were measured before challenge that were found to be lower for IgG3 and IgG1–H435R than for IgG1 and IgG3–R435H ( Fig. 7a ). Bacteremia and pneumonia were determined 24 h later [37] . IgG1 and IgG3–R435H completely protected against bacteremia, whereas IgG3- and IgG1–H435R- treated mice were partly protected ( Fig. 7b ). IgG3–R435H demonstrated a significantly better protection against pneumonia than IgG1 and IgG3, whereas IgG1–H435R was not protective ( Fig. 7c ). A complete clearance for a large fraction of the mice was only observed in the IgG3–R435H-treated group ( Fig. 7b,c ). 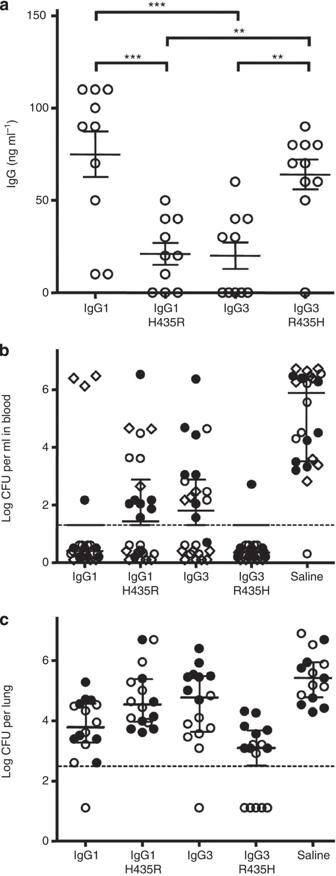Figure 7: H435-containing IgG3 has increased serum persistence in mice and protects against pneumococcal pneumonia. (a) Serum IgG levels 48 h after injecting 1 μg the IgG variants into outbred NMRI mice. IgG1–H435R and IgG3 show lower serum levels than IgG1 and IgG3–R453H. **P≤0.01; ***P≤0.001. (b) Three and (c) two experiments, showing outbred NMRI mice (8–10 per group per experiment) that were passively immunized intraperitoneally with 3 μg (circles symbols) or 1 μg (diamond) recombinant IgG anti-Streptococcus pneumoniae6 or placebo 48 h before challenge with pneumococci of serotype 6A. Results from individual experiments are shown using the same symbol throughout (open or closed circles and diamonds). The number of bacteria found in (b) blood and (c) lungs 24 h after challenge are shown. (b) All but one mouse in the control group developed bacteremia, while all but four mice receiving WT IgG1 and all but one mouse receiving IgG3–R435H were completely protected. Approximately half of the mice receiving either IgG1–H435R or WT IgG3 developed bacteremia. (c) High numbers of bacteria were found in the lungs of control mice. All IgG-treated mice were significantly protected from lung infection, with lowered level of bacterial burden, with few mice in each group completely protected with no detectable bacteria. IgG3–R435H protected the mice significantly better than all other IgG variants, with five mice without detectable lung or blood infection. The dotted lines indicate the level of detection. Data in (a) represent the IgG levels in individual mice together with means and standard errors of means; data in (b,c) represent the bacterial load of individual mice together with medians (assuming the level of detection for individuals without detectable bacteria) and interquartile ranges, statistical comparison is tabulated inTable 1. The statistical analysis of the data in Figure 7b is displayed in Table 1 . Figure 7: H435-containing IgG3 has increased serum persistence in mice and protects against pneumococcal pneumonia. ( a ) Serum IgG levels 48 h after injecting 1 μg the IgG variants into outbred NMRI mice. IgG1–H435R and IgG3 show lower serum levels than IgG1 and IgG3–R453H. ** P ≤0.01; *** P ≤0.001. ( b ) Three and ( c ) two experiments, showing outbred NMRI mice (8–10 per group per experiment) that were passively immunized intraperitoneally with 3 μg (circles symbols) or 1 μg (diamond) recombinant IgG anti- Streptococcus pneumoniae 6 or placebo 48 h before challenge with pneumococci of serotype 6A. Results from individual experiments are shown using the same symbol throughout (open or closed circles and diamonds). The number of bacteria found in ( b ) blood and ( c ) lungs 24 h after challenge are shown. ( b ) All but one mouse in the control group developed bacteremia, while all but four mice receiving WT IgG1 and all but one mouse receiving IgG3–R435H were completely protected. Approximately half of the mice receiving either IgG1–H435R or WT IgG3 developed bacteremia. ( c ) High numbers of bacteria were found in the lungs of control mice. All IgG-treated mice were significantly protected from lung infection, with lowered level of bacterial burden, with few mice in each group completely protected with no detectable bacteria. IgG3–R435H protected the mice significantly better than all other IgG variants, with five mice without detectable lung or blood infection. The dotted lines indicate the level of detection. Data in ( a ) represent the IgG levels in individual mice together with means and standard errors of means; data in ( b , c ) represent the bacterial load of individual mice together with medians (assuming the level of detection for individuals without detectable bacteria) and interquartile ranges, statistical comparison is tabulated in Table 1 . Full size image Table 1 Full size table Collectively, these data reveal that the short half-life described for human IgG3 is due to the arginine in position 435, that can be overcome by introducing an histidine present in this position in the G3m( s , t ) allotypes and other IgG subclasses. The in vivo application of H435–IgG3 combines the properties of long half-life and strong effector functions that surpasses that of human IgG1. In this study, we investigated the binding of IgG3 to FcRn, which, although slightly lower and less pH-dependent, was surprisingly similar to IgG1. In agreement with this, we found FcRn-mediated transport of purified IgG3 to be comparable to that of IgG1. These findings fail to explain the short half-life of IgG3 in humans. However, we found an unexpected inhibition of IgG3 transport in the presence of other IgG subclasses. This was because of intracellular competition for FcRn-mediated transport owing to a single amino acid difference in position 435 between IgG3(arginine) and the other IgG subclasses (histidine), which explains the shorter plasma half-life of IgG3. Mutating this arginine in IgG3 to histidine abrogated the inhibition by IgG1, without affecting the superior effector functions of IgG3. FcRn-mediated transport and degradation were studied in hFcRn-transfected human A375 cells and in the naturally FcRn-expressing human choriocarcinoma cellline JAR. The transport rates of purified IgG1 and IgG3 were similar for various IgG sources. However, in both cell types, the transport of IgG3 was inhibited by addition of IgG1. This inhibition was observed for myeloma IgG1 combined with IgG3 purified from Intramuscular Ig (IMIg), for V-gene-matched recombinant IgGs, and for IVIg in which the inhibition could be alleviated by a protein-A-based inhibitor of FcRn–IgG-binding (Z-domain) specific for IgG1, IgG2 and IgG4. The transport rate was independent of the IgG concentration indicating that an excess of FcRn over IgG will exist early after internalization. However, Ober et al . showed that there is a progressive depletion of FcRn after endo- or pinocytosis events as FcRn-containing vacuoles without IgG are routed away from sorting endosomes containing both IgG and FcRn [15] . Under these circumstances, competition between IgG1 and IgG3 for formation of FcRn–IgG complexes could favour IgG1 binding at low pH (refs 21 , 38 , 39 ). Significant transport inhibition of an excess of IgG3 was observed using very low concentrations of IgG1. Possibly this can be explained by recent findings showing that routing of IgG and FcRn does not take place inside discrete vesicles, but through elongated tubules and/or multiple recycling-endosomes tethered by tubules [13] , [15] , [39] . Here IgG probably binds FcRn in a stochiometry of 1:2, with two FcRn molecules on parallel membranes binding to one IgG molecule [21] , [39] . If IgG in transit goes through multiple checkpoints in tubule-tethered recycling-endosomes [15] , then competition between IgG3 and IgG1 may occur sequentially. Differences in on-rates were the most prominent finding from the interaction kinetics studies, and this may at least partly explain the ability of low concentrations of IgG1 to inhibit IgG3-transport. Our findings that reduced IgG3 transport in the presence of IgG1 coincides with enhanced IgG3 degradation, support the hypothesis that this effect occurs after uptake and within developing lyso- and/or sorting endosomes. We found that mutating position 435 in IgG to an alanine-reduced transport almost to background levels and that IgG1–H435A was unable to inhibit FcRn-mediated IgG3 transport. Transport-inhibition of IgG3 by IgG1 was completely reversed by swapping the amino acids normally present in IgG1 and IgG3 at position 435 (resulting in IgG1–H435R and IgG3–R435H). This strongly indicated that human IgG1 is more adept at FcRn-mediated transport than IgG3, solely because of the R present at position 435 in IgG3. R435-containing IgG also bound shFcRn with a slightly lower affinity than H435-containing IgGs, and soluble IgG1 was better than IgG3 in inhibiting binding of shFcRn to solid-phase immobilized IgG3. This amino acid difference was found to affect IgG3 binding to FcRn in two ways—likely through reduced sensitivity to deprotonation resulting in enhanced binding at pH 7.4, and through steric hindrance, causing decreased binding at pH 6.0, suggesting IgG3 to have a decreased competitiveness for pH-dependent FcRn binding and release, and thus for the overall transport. To study whether our in vitro observations also apply in vivo , we analysed sera from agammaglobulinemic patients who receive regular IVIg replacement therapy that contain both R435- and H435-bearing IgG3 allotypes. We measured the relative IgG subclasses, and IgG3 allotype levels found in IVIg and sera, four weeks after the previous IVIg dose was given. In agreement with our in vitro findings, we found that these sera were enriched for the H435-containing IgG3 allotypes compared with total IgG3, demonstrating that the R435 is also responsible for the lack of competitive FcRn-mediated rescue and short half-life of IgG3 in humans. In accordance with this, we found the serum persistence of IgG1 and IgG3 R435H to be higher than that of IgG3 and IgG1 H435R in outbred NMRI mice. Furthermore, these findings show that the longer hinge of IgG3 does not lead to increased proteolytic degradation, which has been postulated to contribute to the lower half-life of IgG3 (ref. 4 ). IgG3 binds FcγRIII and C1q with higher affinity than IgG1 and is capable of mediating considerably stronger effector functions, such as antibody-dependent cellular cytotoxicity, respiratory burst phagocytosis [1] , [36] , [40] , [41] , [42] , and complement-dependent cytotoxicity towards tumour cells [3] , [43] . This suggests IgG3 containing H435 to be a more effective candidate for in vivo immunotherapies. In an in vivo model of IgG-mediated protection against pneumococcal sepsis and bacteremia WT IgG3 gave comparable protection against pneumonia as IgG1. However, IgG3–R435H protected mice significantly better than either IgG1 or IgG3 against pneumococcal pneumonia, correlating both with its enhanced effector functions and half-life in mice, and confirming its therapeutic potential [24] . In summary, IgG3 is known for both its superior effector functions compared with IgG1—the most commonly used isotype used for immunotherapy—but also for its short in vivo half-life [4] , [5] , [35] , [36] . We now show that FcRn can in fact rescue and transcytose IgG3 as efficiently as IgG1, but not in the presence of the other IgG subclasses. Our data support a model where IgG3 loses competition for FcRn binding and routing away from the lysosomal pathway, explaining its high catabolism in vivo . We demonstrate that this can be resolved by replacing the R435 with a histidine, as is the case in a rare natural variant. The epitope comprising the H435 in G3m( s , t ) is an isoallotype that is found in all other IgG subclasses, and its detectable presence in IVIg has not been documented to cause adverse reactions in patients. The extended half-life of the IgG3–R435H variant has important implications for current and future antibody-based therapies aimed at achieving maximal effector functions. Cell culture Human choriocarcinoma cells (JAR, ATCC, VA) were grown in IMDM medium (Cambrex) and melanoma cells (A375, FcRn − β2m + , ATCC) in RPMI 1,640 medium (Invitrogen/Gibco), both supplemented with l-glutamin (300 μg ml −1 , Invitrogen), penicillin (100 U ml −1 , PAA Laboratories), streptomycin (100 μg ml −1 , PAA) and 10% foetal calf serum (FCS). A375–FcRn Human FcRn messenger RNA was amplified after first strand cDNA synthesis by PCR using the forward 5′-GGATCCACCATGGGGGTCCCGCGGCCTCAGC-3′ and reverse 5′-GAATTCTCAGGCGGTGGCTGGAATCAC-3′ primers and ligated into pGEM-T (Promega, Madison, WI, USA). The Bam HI– Eco RI fragment was subcloned into the pMX-puro vector (DNAX) and transfected together with a packaging vector into 293T-cells [44] . Supernatants were used to transduce A375 cells [45] . Expression of FcRn was confirmed by quantitative RT–PCR [17] . IgG IVIg was obtained from Sanquin. Pooled myeloma IgG1 was purified from three multiple myeloma patients by serum protein precipitation and depletion of other subclasses by sephadex-bound anti-subclass Ig. IgG3 was obtained from IMIg (Sanquin) after depleting other IgG with protein A. Recombinant IgG1, IgG3 and IgG1–H435A have been described before [17] , [37] . Recombinant IgG were produced in 293 Freestyle cells (Invitrogen) according to the manufacturer's instructions, and purified using HiTrap protein A (for H435-containing IgGs) or protein G using the Acta Prime Plus system (GE Healthcare). IgG1–H435R, IgG3–R435A and IgG3–R435H were generated using the Quickchange Site-directed-mutagenesis kit (Stratagene) with the following and reverse complementary oligonucleotide primers: IgG1–H435R:: GAGGCTCTGCACAACC G CTACACGCAGAAGAGCC IgG3-R435A:: GAGGCTCTGCACAAC GC CTACACGCAGAAGAGCC IgG3–R435H:: GAGGCTCTGCACAACC A CTACACGCAGAAGAGCC All mutations were confirmed by sequencing before expression. The endotoxin levels of the various batches was tested and confirmed to be very low or absent by measuring IL-6 production of monocyte-derived immature DC, as described in ref. 46 . Z domain The gene encoding the Z-domain was amplified by PCR from the vector pThio-His-ZZ [47] using 5′-GGATCCGTAGACAACAAATTCAAC-3′ (forward) and 5′-CTGCAGTTATTTCGGCGCCTGAGCATC-3′ (reverse), and cloned into pGEM-T (Promega). The Bam HI– Not I fragment was cloned into the pGEX 6.2 expression vector and expressed in Escherichia coli . The GST tag was removed using PreScision protease (GE healthcare) and the Z-domain eluted off the glutathione sepharose 4B column (GE healthcare) by gravity flow and dialysed against PBS. IgG transcytosis 12 mm polycarbonate Transwell filters (0.4 μm pore size, Costar/Corning) were inoculated with 5×10 5 cells, grown overnight to confluence, washed with PBS and medium replaced with fresh 1.5 ml medium basolaterally and 0.5 ml apically (IMDM at pH 7.4 with supplements as stated above). Mixtures of IgG contained 125 pg ml −1 streptavidin-HRP (Sanquin) to assess background transport. Apical to basolateral transport was calculated according to ([IgG] basolateral ×1.5 ml)/([IgG] input ×0.5 ml)×100%. All experiments were performed in triplicate. Surface plasmon resonance assays All experiments were performed using a Biacore 3000 instrument, CM5 biosensor chips and amine coupling as described by the manufacturer (GE Healthcare). Injections were done using phosphate buffer (67 mM phosphate buffer, 0.15 M NaCl, 0.05% Tween20) at pH 6.0. Kinetic evaluations were performed using immobilized shFcRn–GST ( ∼ 1,000 RU) [48] , [49] , and IgG variants (2–500 nM) injected. Alternatively, IgG was immobilized ( ∼ 1,500 RU) and shFcRn injected (7–4,000 nM). For the competitive SPR assay, chips were coupled with IgG ( ∼ 1,300 RU) and shFcRn (100 nM) was injected alone or together with serial dilutions of IgG1 or IgG3. Binding at different pH was done in a phosphate buffer with 500 nM IgG injected over immobilized shFcRn ( ∼ 2.000 RU). All experiments took place at 20–60 μl min −1 , 25°C, and HBS-P buffer (GE Healthcare) at pH 7.4 was used for regeneration. Binding analyses were performed using the BIAevaluation wizard software 4.1. Agammaglobulinemia patients Serum samples from three agammaglobulinemia patients, taken 4 weeks after receiving IVIg, were assessed for IgG subclass levels which were expressed as relative IgG concentrations compared with that found in IVIg (Relative IgG levels at week 4 (%)=[IgG S ] W4 /[IgG T ] W4 /([IgG S ] IVIg /[IgG T ] IVIg )×100%, where W4 stands for serum at week 4 after IVIg injection, S for Subclass and T for Total). Serum samples were anonymous rest material acquired during routine IgG-evaluation of these patients, and, therefore, did not require a Medical Ethical Committee evaluation according to the institutional Committee of the Academic Medical Centre of the University of Amsterdam. IgG quantification IgG subclass concentrations in sera were determined by Nephelometry (Behringer Nephelometer II, Behringer diagnostics). For other experiments, IgG concentrations were determined by sandwich ELISA using subclass specific mouse monoclonal antibodies (IgG1:MH161-1; IgG3:MH163-1, Sanquin) or allotype-specific monoclonal anti G3m( s , t ) [32] (1.5A10, Sanquin, Supplementary Fig. S4 ) for capture. Mouse-anti-IgG-HRP (Southern Biotech) was used for detection in all assays except the G3m( s , t ) ELISA where mouse anti-IgG3-HRP (MH163-1, Sanquin) was used. Concentration was read of standard curves made using the same IgG preparations used for transport or to treat patients. Passive protection The pneumococcal infection model has been described before [37] , [50] . In brief, outbred NMRI mice (Taconic) were passively immunized intraperitoneally with 3 μg of recombinant IgG (diluted in 200 μl PBS) or saline only, 48 h before challenge with a virulent pneumococcal strain of serotype 6A. Mice were anesthetized and challenged intranasally with 2×10 7 CFU pneumococci in 50 μl sterile 0.9% saline. Twenty-four hours after challenge, the mice were killed and bacterial load evaluated by colony counting as described in refs 37 , 50 . All in vivo studies complied with the Animal Experimental Committee of Iceland According to the Act on Animal Welfare no 15/1994. Statistical analysis and data sets All data represent the mean and standard deviation of at least three independent experiments. All transcytosis assays consisted of three replicates. GraphPad Prism version 4.00 for Windows (GraphPad Software) was used for all statistical analysis. Significance was set at P ≤0.05, and the level of significance is indicated on all figures as * P ≤0.05; ** P ≤0.01; *** P ≤0.001. How to cite this article: Stapleton, N. M. et al . Competition for FcRn-mediated transport gives rise to short half-life of human IgG3 and offers therapeutic potential. Nat. Commun. 2:599 doi: 10.1038/ncomms1608 (2011).